Ion transport controlled by nanoparticle-functionalized membranes From proton exchange membranes in fuel cells to ion channels in biological membranes, the well-specified control of ionic interactions in confined geometries profoundly influences the transport and selectivity of porous materials. Here we outline a versatile new approach to control a membrane’s electrostatic interactions with ions by depositing ligand-coated nanoparticles around the pore entrances. Leveraging the flexibility and control by which ligated nanoparticles can be synthesized, we demonstrate how ligand terminal groups such as methyl, carboxyl and amine can be used to tune the membrane charge density and control ion transport. Further functionality, exploiting the ligands as binding sites, is demonstrated for sulfonate groups resulting in an enhancement of the membrane charge density. We then extend these results to smaller dimensions by systematically varying the underlying pore diameter. As a whole, these results outline a previously unexplored method for the nanoparticle functionalization of membranes using ligated nanoparticles to control ion transport. Transport and selectivity in membrane-based separation processes are controlled by a combination of chemical-, charge- and size-based interactions, which in turn must be controlled with the utmost precision to optimize performance. For naturally occurring systems such as biological membranes, the well-regulated control of mass and ion transport is accomplished through highly specialized protein channels of nanometre- and subnanometre-sized dimensions, capable of displaying extraordinary degrees of transport and efficiency [1] , [2] . For example, ion channels such as the KcsA channel can selectively transport potassium ions 1,000 times more readily than identically charged and similarly sized sodium ions [2] . Attempts to achieve this degree of control in synthetic systems and other applied technologies are dependent upon controlled synthesis techniques or alternate pathways towards further functionalization of porous materials [3] , [4] , [5] . In industrial-based applications, such as reverse osmosis (RO) membranes for desalination, detailed interfacial polymerization techniques and a combination of reactants for the active layer of thin-film composite membranes are required to simultaneously achieve a particular membrane morphology or pore size with a desired set of chemical interactions to influence transport [6] , [7] . Such efforts have reached a considerable level of maturity [8] , [9] ; however, recent efforts to further functionalize these systems using nanoparticles (NPs) [10] , [11] highlight the underlying fact that further improvements can be made. Despite significant differences over a wide range of length scales, these and other membrane-based-separation processes including those found in emergent technologies composed of gold [12] , carbon [13] , [14] and boron nitride [15] nanotubes, as well as porous silicon [16] and graphene [17] , all depend on the well-specified control of molecular interactions in confined geometries. An example of particular interest is the role of electrostatics and the effective charge density of a membrane’s pore. Charge-based effects can influence transport at length scales many times the size of the ion and form the basis of many ionic separation processes [18] . One of the key features for the development of model systems to capture the essential physics and chemistry of the process, which in turn can be used to generate a set of design principles to optimize a membrane’s ionic separation performance, is the ability to independently control charge-based interactions for a given membrane morphology, either during the synthesis process itself or in additional steps of functionalization [19] . Here we describe a new approach to achieve these goals using films of densely packed colloidal NPs to control transport. NPs are functionalized a priori by a suitable choice of encapsulating ligand chemically adsorbed to the NP surface and subsequently deposited on commercially available porous polycarbonate (PC) substrates. When deposited on the substrate, the encapsulating ligands of the NPs serve two important purposes that provide an effective and convenient means to functionalize a porous substrate and influence transport. First, ligand–ligand interactions, aided by ligand interdigitation, enable a stable film over a wide range of ionic solutions and pH conditions. Second, for any uncovered pore on the substrate, ligands attached to the particles deposited at the pore entrance act to modify the interfacial region of the pore and provide a means to deliver chemical functionality to that pore through carefully selected terminal functional groups. We use these two features to generate a functionalization scheme that is largely substrate-independent and retains the functionality of individual components. When compared with other membrane technologies, the resulting NP-functionalized membranes show a number of desirable features such as high-flux characteristics and a large degree of versatility in engineering a desired set of interactions. Here we demonstrate that these interactions can be specifically tailored to influence ionic transport. Such behaviour opens up new possibilities where ligated NPs are functionalized a priori with the desired molecular species, serving as building blocks for delivering some desired chemical functionality, which in turn could be used to generate membrane-active layers of arbitrary thicknesses or even alternating composition. Assembly of NP-functionalized membranes Herein, we study the behaviour of colloidal gold-core NPs (AuNPs) ~5.5 nm in diameter encapsulated by a monolayer shell of alkanethiol ligands. Our approach of NP functionalization is schematically illustrated in Fig. 1a–d . NP films were prepared by sequentially depositing monolayers of AuNPs using a slightly modified procedure from what we have used previously to form free-standing NP monolayers of various core materials and encapsulating ligands [20] , [21] , [22] , [23] (see Methods). Briefly, NP monolayers were draped one monolayer at a time onto the PC substrate, and the process repeated until a desired number of transfers were obtained. When deposited on the PC substrate, NP monolayers adhere exceedingly well, which we associate with hydrophobic forces between the ligands and the polyvinylpyrrolidone coating of the PC substrate [24] . Subsequent layers adhere to one another through ligand interdigitation and van der Waals forces [25] , [26] , leading to stable NP films over a wide range of ionic solutions and conditions. Here the NP film is transferred to the underlying PC substrate while leaving a sufficient fraction of the pre-existing pores uncovered as verified by scanning electron microscopy (SEM) analysis. Once assembled, the AuNP-modified PC substrates (hereafter referred to as membranes) were incorporated into a peristaltic pump system, and ionic solutions were continuously flowed over the membrane (feed solution), while the volume passing through the membrane (permeate) was collected. Owing to the high-flux characteristics, with measured membrane permeabilities on the order of L p ~(10 −9 –10 −10 ) m s −1 Pa −1 , the pump alone was sufficient to drive a measurable flow through the NP-modified membrane while simultaneously acting to remove any concentration polarization effects. Conductivity was measured for both the feed and permeate solutions to quantify the ion rejection capacity of the membranes. 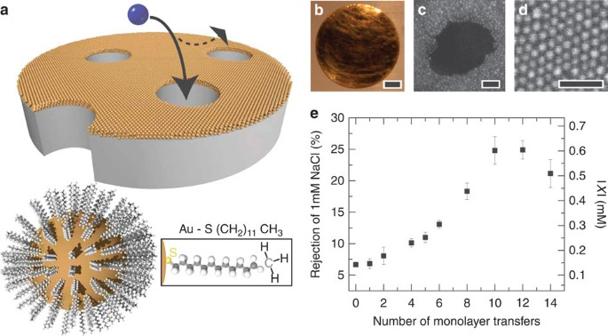Figure 1: Nanoparticle-modified membranes. (a) Schematic of a AuNP film deposited on a porous PC substrate and subsequent transport pathway for an electrolyte (blue sphere) moving through an uncovered pore. Ligands absorbed to the surface of the AuNPs modify the pore entrance and set the chemistry of the underlying pore through the ligand terminal group; as shown methyl-terminated dDT. (b) Optical image of a dDT–AuNP-modified PC substrate, 13 mm in diameter, after 12 × monolayer transfers (scale bar 2 mm). (c) SEM of a single uncovered 100-nm pore and (d) the dDT–AuNP film (scale bars inc,d25 nm). (e) Electrolytic transport properties of dDT–AuNP-modified PC substrates for 1 mM NaCl. Conductivity rejection (leftyaxis) and corresponding membrane charge density (rightyaxis), as calculated in the Donnan model, equation (1), are shown as a function of the number of dDT–AuNP monolayers transferred to the underlying substrate. Error bars represent s.d.’s in individual measurements of the conductivity rejection; on average, six measurements were made for each monolayer transfer. As additional monolayers are transferred to the substrate, the rejection approaches a saturating value of ~25%, which we associate with the maximum rejection of methyl-terminated AuNP membranes, given an underlying pore diameter of 100 nm. Figure 1: Nanoparticle-modified membranes. ( a ) Schematic of a AuNP film deposited on a porous PC substrate and subsequent transport pathway for an electrolyte (blue sphere) moving through an uncovered pore. Ligands absorbed to the surface of the AuNPs modify the pore entrance and set the chemistry of the underlying pore through the ligand terminal group; as shown methyl-terminated dDT. ( b ) Optical image of a dDT–AuNP-modified PC substrate, 13 mm in diameter, after 12 × monolayer transfers (scale bar 2 mm). ( c ) SEM of a single uncovered 100-nm pore and ( d ) the dDT–AuNP film (scale bars in c , d 25 nm). ( e ) Electrolytic transport properties of dDT–AuNP-modified PC substrates for 1 mM NaCl. Conductivity rejection (left y axis) and corresponding membrane charge density (right y axis), as calculated in the Donnan model, equation (1), are shown as a function of the number of dDT–AuNP monolayers transferred to the underlying substrate. Error bars represent s.d.’s in individual measurements of the conductivity rejection; on average, six measurements were made for each monolayer transfer. As additional monolayers are transferred to the substrate, the rejection approaches a saturating value of ~25%, which we associate with the maximum rejection of methyl-terminated AuNP membranes, given an underlying pore diameter of 100 nm. Full size image Methyl-terminated AuNP membranes For PC substrates modified with AuNPs encapsulated by methyl-terminated dodecanethiol ligands (dDT-AuNPs), the transport of electrolytes depends on a variety of parameters, including the number of monolayer transfers, electrolyte concentration and pH of the feed solution. Shown in Fig. 1e is a representative conductivity rejection for 1 mM sodium chloride (NaCl) as a function of the number of dDT-AuNP monolayers transferred to the PC substrate. The rejection increases before stabilizing to a constant value (~25%), independent of both the number of monolayer transfers and flow rate. As additional monolayers are added, the thickness of the NP film increases linearly with each monolayer deposition, as shown by atomic force microscopy measurements (see Supplementary Fig. 1 ). During the process, some pores are covered, which results in a drop in flow rate. For suitably prepared membranes, rejection values were identical over two orders in magnitude in flow rate. We infer because of the behaviour at saturation that transport is dominated by uncovered pores and that a minimum number of transfers is required to modify the pore openings of the underlying substrate with a sufficient thickness of the NP film. Because the ion transport is dominated by flow through large uncovered pores (~100 nm in diameter), steric hindrance effects are not significant [27] , [28] and ions can go through the pores without much retardation [5] , so that we can describe our system using the Donnan theory for membrane equilibria [29] . In the Donnan model, the rejection, R , of an ionic species is controlled by the charge density of the membrane via [30] where c F and c p are the concentration of co-ions in the feed and permeate solutions, X is the membrane charge density, the subscripts i and j refer to co- and counterions, and z is the ion valence. In the context of Donnan exclusion, the maximum ~25% rejection of 1 mM NaCl for methyl-terminated dDT-AuNP-modified membranes corresponds to a membrane charge density | X |≈0.6 mM. It is possible that thiol binding to gold surfaces through the formation of thiolate could cause the NP surface to be partially negatively charged, as shown in the electrophoretic measurements in ref. 31 . However, it is also possible that charge develops because of the adsorption of ions from solution [32] . Motivated by previous studies of methyl-terminated alkanethiols on Au metallic films, which associated the adsorption of residual OH − ions to the development of a negative charge [33] , we investigated the rejection of 1 mM ionic solutions varying in their native pH ( Fig. 2 ). The resulting trend illustrates a rejection increase in more basic solutions, in which | X | can vary by a factor of 3 as the pH changes from ~6 to ~9 (| X |=0.35–1.1 mM). Such behaviour supports OH − adsorption as the underlying mechanism for the development of a negative charge density. It also highlights an appealing feature of methyl-functionalized membranes in the context of pH-responsive porous materials. Membranes of this type showed no hysteresis between salt runs (as verified by comparing 1 mM NaCl in between each of the runs), demonstrating the stability of NP-modified membranes over a range of acidic and basic conditions (pH=3–11 in our experiments). Moreover, these observations suggest that interactions can be controlled by the ligand terminal group and engineered accordingly. 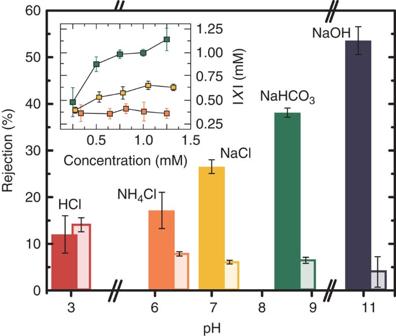Figure 2: Conductivity rejections and pH sensitivity of methyl-terminated nanoparticle membranes. Rejection sequences for methyl-terminated dDT-AuNP-modified PC membranes (solid bars, dark shading) and the bare PC substrate alone (light shading) are shown for 1 mM solutions of acidic (HCl and NH4Cl), neutral (NaCl) and basic (NaHCO3and NaOH) salts as a function of their natural pH. The pH of NH4Cl (~6.2) and NaHCO3(~8.7) were calculated using equilibrium constants ofKb=1.8 × 10−5andKb=2.25 × 10−8, respectively, while the pH of HCl, NaCl and NaOH were taken as 3, 7 and 11, respectively. Error bars correspond to s.d.’s in individual measurements of the conductivity rejections; on average, six measurements were made for each electrolyte. Comparing the rejection of the bare underlying PC substrate alone with that of the composite dDT–AuNP membrane, the membrane has become neutralized or even positively charged at low pH~3 (HCl), while at high pH~11 (NaOH), a more saturated adsorption of OH−ions leads to the large conductivity rejection. Inset: calculated membrane charge densities using the Donnan model, equation (1), over a range of concentrations for NH4Cl, NaCl and NaHCO3with limiting values of 0.35, 0.6 and 1.1 mM, respectively. Figure 2: Conductivity rejections and pH sensitivity of methyl-terminated nanoparticle membranes. Rejection sequences for methyl-terminated dDT-AuNP-modified PC membranes (solid bars, dark shading) and the bare PC substrate alone (light shading) are shown for 1 mM solutions of acidic (HCl and NH 4 Cl), neutral (NaCl) and basic (NaHCO 3 and NaOH) salts as a function of their natural pH. The pH of NH 4 Cl (~6.2) and NaHCO 3 (~8.7) were calculated using equilibrium constants of K b =1.8 × 10 −5 and K b =2.25 × 10 −8 , respectively, while the pH of HCl, NaCl and NaOH were taken as 3, 7 and 11, respectively. Error bars correspond to s.d.’s in individual measurements of the conductivity rejections; on average, six measurements were made for each electrolyte. Comparing the rejection of the bare underlying PC substrate alone with that of the composite dDT–AuNP membrane, the membrane has become neutralized or even positively charged at low pH~3 (HCl), while at high pH~11 (NaOH), a more saturated adsorption of OH − ions leads to the large conductivity rejection. Inset: calculated membrane charge densities using the Donnan model, equation (1), over a range of concentrations for NH 4 Cl, NaCl and NaHCO 3 with limiting values of 0.35, 0.6 and 1.1 mM, respectively. Full size image Carboxyl- and amine-terminated AuNP membranes To investigate charged groups more typical to those found in nanofiltration and RO membranes [3] , [6] , [7] , we studied the behaviour of PC substrates modified with AuNPs containing carboxyl- and amine-terminated ligands with alkane chain lengths similar to their dDT counterparts. Ligand modification was carried out either before each monolayer deposition or after a certain thickness of film had been reached (see Methods). The corresponding rejection of the mixed valence salts MgCl 2 , NaCl, and Na 2 SO 4 is shown in Fig. 3 . Similar to the case of methyl-, the charge of carboxyl-terminated ligands is negative as demonstrated by a rejection in the order of R (MgCl 2 )< R (NaCl)< R (Na 2 SO 4 ) [30] . While in the case of methyl, charge is due to OH − adsorption, carboxyl is inherently negative under identical electrolyte conditions due to deprotonation and | X | can be as much as two to three times larger for a given set of ions ( Fig. 3b ). Differences in | X | are related to both the nature of the interaction between ions and the ligand terminal group, as well as the number of active charged sites (for example, the ligand density). In the case of amine, the tendency for protonation drives X to positive values, and the rejection sequence of mixed valence salts switches with respect to methyl- and carboxyl-terminated membranes, resulting in R (MgCl 2 )> R (NaCl)> R (Na 2 SO 4 ) [30] . Given that the primary difference in the ligands is the charge state of the terminal group, we conclude that the dominant interaction for determining transport is the electrostatic interaction between the ligand and ions in solution. 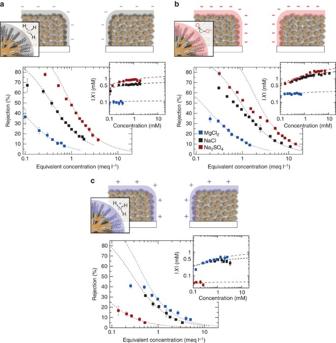Figure 3: Engineering the ligand terminal group to tune the membrane charge. Schematics and measured conductivity rejections for (a) methyl-, (b) carboxyl- and (c) amine-terminated ligands of AuNP-functionalized membranes. Conductivity rejections are shown as function of equivalent electrolyte concentration for mixed valence salts MgCl2(blue), NaCl (black) and Na2SO4(red). Dashed lines represent fits from the Donnan exclusion model, equation (1), under the assumption of a fixed membrane charge density, |X|. Deviations to the model are most prevalent at low electrolyte concentration, resulting from the fact that |X| is not a constant, but depends on the electrolyte concentration as shown in the inset. Insets: absolute magnitude of the membrane charge density calculated from equation (1) plotted as function of electrolyte concentration,cF. Dashed lines represent fits to an empirical equation34,, where A and B are fitting parameters andXeffis identified as an effective charge density. It follows that the membrane charge density scales asfor low electrolyte concentrations, in accordance with Gouy–Chapman theory for weakly charged surfaces32, and becomes independent of feed concentration asXeff→A/Bat large concentrations. The saturation value in charge density, with no explicit feed concentration dependence, was identified previously with the fixed membrane charge density34and is the value used in the overlays for the main figures. Figure 3: Engineering the ligand terminal group to tune the membrane charge. Schematics and measured conductivity rejections for ( a ) methyl-, ( b ) carboxyl- and ( c ) amine-terminated ligands of AuNP-functionalized membranes. Conductivity rejections are shown as function of equivalent electrolyte concentration for mixed valence salts MgCl 2 (blue), NaCl (black) and Na 2 SO 4 (red). Dashed lines represent fits from the Donnan exclusion model, equation (1), under the assumption of a fixed membrane charge density, | X |. Deviations to the model are most prevalent at low electrolyte concentration, resulting from the fact that | X | is not a constant, but depends on the electrolyte concentration as shown in the inset. Insets: absolute magnitude of the membrane charge density calculated from equation (1) plotted as function of electrolyte concentration, c F . Dashed lines represent fits to an empirical equation [34] , , where A and B are fitting parameters and X eff is identified as an effective charge density. It follows that the membrane charge density scales as for low electrolyte concentrations, in accordance with Gouy–Chapman theory for weakly charged surfaces [32] , and becomes independent of feed concentration as X eff → A/B at large concentrations. The saturation value in charge density, with no explicit feed concentration dependence, was identified previously with the fixed membrane charge density [34] and is the value used in the overlays for the main figures. Full size image Functionalized AuNP membranes The results outlined above demonstrate that encapsulating ligands of NPs can be used to control transport through a suitable choice of ligand functional terminal groups. Another appealing feature is the possibility of subsequent functionalization of the ligated NPs by exploiting a known binding affinity. To demonstrate this, we employed surface coupling chemistry to compare | X | before and after functionalizing carboxyl-terminated membranes with a highly charged carboxyl-specific dye (see Methods). Owing to the dye’s three negatively charged sulfonate groups, | X | should increase by threefold if all available sites on the membrane were populated; however, over a range of different reaction and binding conditions, dye-conjugated carboxyl membranes reproducibly increased | X | only by a factor of ~2, | X before |=1.1±0.1 mM and | X after |=2.2±0.1 mM. We propose that electrostatic repulsions between incoming dye molecules and those already bound to the surface, as well as steric constraints imposed by incorporating this relatively large dye molecule, prevent a fully conjugated surface. Nevertheless, such data clearly demonstrate the general principle of further functionalization of the ligand terminal group. Variation of the underlying pore diameter In purely charge-based separation processes, the absolute magnitude of the membrane charge controls the degree of response. Given that the average number of ligands on each NP surface has a fixed value, the amount of surface charge density, σ , each particle can develop is ultimately limited by the packing fraction of ligands on the NP surface. However, at fixed surface charge density, the effective membrane charge density | X | will increase with decreasing pore diameter 2 r , as described by a simple scaling relationship [34] , where F is the Faraday constant. Fig. 4 shows | X | for carboxyl-terminated membranes over a range of different pore diameters (15–800 nm). Overall, we find a reasonably good agreement with equation (2). Some deviations from the 1/ r dependence, especially for smaller pores, could come from several factors. First, during the deposition of NP films, a fraction of the pores get covered, the number of which increases as additional layers are added, leading to a reduction in flow rate. As the pore diameter of the underlying substrate decreases, so does its flow rate. With each additional deposition of AuNPs, the overall flow rate of the composite membrane can reach values too small to be probed in the present pump-based system before reaching saturation, biasing the measurement to lower | X | values (see Fig. 1e ). Second, the assumption of a fixed surface charge density is critically dependent on the extent of carboxyl ligand replacement. Carboxyl-terminated membranes were fabricated by modifying pre-existing methyl-terminated dDT-AuNP membranes in the presence of ethanol (see Methods). Under these conditions, we do not expect the introduction of carboxyl-terminated ligands to displace the already bonded methyl ligands on the NP surface. Therefore, there is most likely a mixed population of ligands, and the extent of ligand replacement may vary slightly for different samples, resulting in a variation of the membrane charge density. In addition, the presence of pores that are partially covered and thus have a smaller effective size could inflate the charge density extracted from the measurements. Lastly, some deviations from a 1/ r scaling could come from the assumption of a purely Donnan-based rejection mechanism, which would explain deviations at smaller pore sizes [27] , [28] , [29] , [34] . At large pore sizes, especially for the bare PC substrates, we believe sample-to-sample and measurement uncertainties are responsible. In both cases, a nonlinear fit may be appropriate; however, we believe these deviations are not significant enough to do so. Under the identification of a 1/ r scaling, the observed values for | X | are in agreement with studies of carboxyl-terminated alkanethiols on planar metallic (Au) films under the assumption of equivalent ligand surface coverage, and therefore fixed surface charge densities [33] . Averaging over all measured charge densities ( Fig. 4 ) and rescaling by the pore diameter, we find σ =0.20±0.08 μC cm −2 . Extrapolating to pore sizes on the order of a nanometre, these measurements indicate that carboxyl-terminated NP membranes exhibit a charge density that compares well with the polyamide-active layer of thin-film composite membranes [11] , while at larger length scales (for example, 100 nm), the corresponding rejections exceed that of carbon nanotubes [13] , [14] . 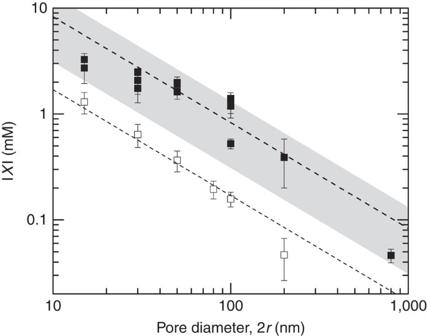Figure 4: Inverse pore diameter scaling. Membrane charge density in the presence of NaCl for carboxyl-terminated AuNP-modified PC membranes (filled symbols) and bare PC substrates alone (open symbols) as a function of the substrate pore diameter, 2r. For the bare PC membranes, each point represents the average of two to three individual experiments using different substrates. For AuNP-modified membranes, each point represents a different membrane, and error bars correspond to s.d.’s in the average charge density obtained over a range of different sodium chloride concentrations where the membrane charge density becomes independent of feed concentration. The lines represent best fits assuming a 1/(2r) scaling for the underlying PC substrate (thin dashed line) and the nanoparticle-functionalized membranes (thick dashed line). The shaded area denotes a representative scaling region for the range of measured charge densities. Figure 4: Inverse pore diameter scaling. Membrane charge density in the presence of NaCl for carboxyl-terminated AuNP-modified PC membranes (filled symbols) and bare PC substrates alone (open symbols) as a function of the substrate pore diameter, 2 r . For the bare PC membranes, each point represents the average of two to three individual experiments using different substrates. For AuNP-modified membranes, each point represents a different membrane, and error bars correspond to s.d.’s in the average charge density obtained over a range of different sodium chloride concentrations where the membrane charge density becomes independent of feed concentration. The lines represent best fits assuming a 1/(2 r ) scaling for the underlying PC substrate (thin dashed line) and the nanoparticle-functionalized membranes (thick dashed line). The shaded area denotes a representative scaling region for the range of measured charge densities. Full size image In this article, we have outlined two distinct approaches to tune the membrane charge density by varying the inherent charge of the ligand terminal group itself and incorporating surface coupling chemistry to further modify the terminal group charge state. We then utilized a simple scaling argument to extend these results to pores of smaller dimensions. In all cases examined, modification of the porous substrates using ligated NPs reduced the permeabilities only by a small fraction of the original permeability of the bare porous substrate. The corresponding permeabilities of the composite NP-functionalized membranes, L p ~(10 −9 –10 −10 ) m s −1 Pa −1 , are among the highest recorded to date for emergent ion-separation membrane technologies [9] . From a practical perspective, in addition to high-flux characteristics, these results can be applied to much larger substrates and scaled up accordingly. Here the method for NP deposition relied on using a typical water drop of 3 ml to immerse 13-mm-diameter substrates (see Supplementary Fig. 2 ). However, the same method can be applied to much larger interfaces depending on the substrate size and even suitably sized Langmuir–Blodgett troughs for more typical industrial-scale substrates. Moreover, by nature of the assembly, films of particular thickness, with potentially different functionalities encoded into each one of the layers, can be fabricated with relative ease. Perhaps most importantly, we have demonstrated a desirable and readily attainable feature of specifically tailoring transport through a suitable choice of encapsulating ligand chemically absorbed to the NP surface. In this regard, we are able to achieve a desired functionality in a manner similar to, but distinctly different from, those using self-assembled monolayers (SAMs) [35] , [36] , [37] , [38] , [39] , [40] , [41] , which have received considerable attention for a wide variety of applications, including fuel cells [37] and biosensors [42] . In approaches based on SAMs, chemical interactions are engineered into pre-existing porous substrates by utilizing a favourable surface chemistry to bind a monolayer of functionalized molecules. Here by utilizing particles encoded a priori with the desired functionality, we are able to bypass the requirement of a favourable surface chemistry in order to bind the molecules to the surface of the porous substrate itself, or any additional steps coating the substrate with a metal such as gold [38] , [39] , [40] , [41] . Owing to the flexibility by which ligated NPs can be synthesized, including both the core materials themselves and the encapsulating ligands [43] , [44] , we believe the approach outlined here can be generalized to a similar set of functionalities as their SAM counterparts for different core materials. Previous work has already demonstrated that strong ligand–ligand interactions required for NP film stability are attainable not only for alkanethiol-AuNPs [20] , [21] , [22] , [45] , [46] , but other core materials such as cobalt oxide and iron oxide with oleylamine and oleic acid ligands [21] , as well as DNA-coated NPs [47] . The end result is a potentially powerful route towards engineering a set of desired interactions in which colloidal NPs are functionalized a priori with the desired functionality [48] , [49] . In short, ligated NPs serve as fully functionalized building blocks for a type of bottom-up assembly for the active layer of membranes. By extension, successive deposition of ligated NP films opens up exciting possibilities including the fabrication of composite layers, each with a specific chemical function. NP synthesis NPs were synthesized following a well-established digestive ripening technique [50] . Briefly, 208 mg of didodecyldimethylammonium bromide (DDAB) was dissolved into 20 ml of distilled toluene and added to 68 mg of gold chloride (AuCl 3 ), and then sonicated for 15 min. Separately, a 9.4M sodium borohydride (NaBH 4 ) solution in H 2 O was made and left to sit for 8–9 min before adding 72 μl to the DDAB–AuCl 3 solution, which was then stirred for 1 h. Next, 1 ml of dodecanethiol (dDT—HS (CH 2 ) 11 CH 3 ) was added to each 10 ml of the stirred DDAB–AuCl 3 –NaBH 4 solution split into two vials. Then, 20 ml of ethanol was added to each vial to precipitate the particles. The precipitated particles were dried under vacuum and dissolved in 10 ml of distilled toluene. Next, 1 ml of dDT was added and the solution was heated under reflux for a minimum of 4 h. After cooling down, the supernatant was precipitated twice in ethanol to remove synthesis byproducts. The final precipitate was dried under vacuum and re-dispersed in 10 ml of distilled toluene. The NPs were characterized by transmission electron microscopy, showing an average Au core diameter of ~5.5 nm. NP monolayer assembly and deposition PC substrates (Isopore) with nominal pore diameters of 100 nm were purchased from Millipore. For pore diameter studies (for example, Fig. 4 ), substrates were purchased from SPI Supplies, with nominal pore diameters in the range 15–800 nm. According to the manufacturer’s data, all membranes are coated with polyvinylpyrrolidone as a wetting agent. To deposit AuNPs on the surfaces, a PC substrate was placed on chemically resistant Bytac (Saint Gobain Performance Plastics) in a concave Petri dish and completely immersed in distilled water (~3 ml). Subsequently, ~40 μl of a toluene solution containing dDT–AuNPs was added to the three-phase contact line of the water droplet. Under these conditions, the insolubility of water and the dDT–AuNP toluene solution drives the formation of NP monolayers at the air–water interface, which can then be subsequently transferred to different substrates [20] , [21] , [22] , [23] . Here immediately after the toluene evaporated (~10 min), the monolayer was gently draped on the PC membrane by simultaneously tilting the Petri dish and removing the water via a pipette. After deposition, the monolayer was allowed to dry for ~1 h, and then tested for the rejection of 1 mM NaCl. For each membrane studied, additional layers were added to the dDT-AuNP—PC composite membrane by repeating this process until the maximum rejection for 1 mM NaCl was achieved (~25%, Fig. 1e ). Typically, the maximum rejection for 1 mM NaCl was achieved in 6–10 transfers. Ligand modification The following ligands were used for the assembly of carboxyl and amine membranes, respectively: 11-Mercaptoundecanoic acid (HS (CH 2 ) 10 COOH) and 11-Amino-1-undecanethiol (HS (CH 2 ) 11 NH 2 ). The assembly of carboxyl- and amine-terminated membranes were initiated in two different ways that led to equivalent results. First, before transferring dDT–AuNP monolayers to the PC substrates, 2 μl of 75 mM solutions of either carboxyl- or amine-terminated ligands dissolved in ethanol were added to the underlying water containing a dDT–AuNP monolayer at the air–water interface. As the ethanol solution containing the ligands diffused through the droplet, ligands attached to the side of the NP surface in contact with the water. The reaction diffusion process was allowed to continue for ~30 min until a noticeable change in the monolayer colour occurred (sky blue to purple). Binding of ligands to the NP surface was inferred using X-ray analysis and a shift in the first-order diffraction peak (data not shown). Once modified, NP monolayers were transferred on the PC substrates by gently placing the PC substrate in contact with the monolayer at the air–water interface. The process was repeated until a desired number of transfers were obtained. Monolayers were stamped to ensure that the ligand-modified surface was exposed to the ionic solution when assembled into the housing unit. Before taking data, membranes were flushed in a peristaltic pump system using water to remove any unbound ligands, and the conductivity was monitored until a baseline conductivity reading (2–4 μS cm −1 ) was obtained. In a second approach, dDT–AuNP membranes were modified in situ after being assembled on the PC substrates by immersing a native dDT–AuNP membrane in ~600 μl of H 2 O and adding 2 μl of 75 mM solutions of either carboxyl- or amine-terminated ligands suspended in ethanol. The reaction was allowed to proceed for ~30 min. In all cases, repeated flushing with water using the peristaltic pump was used to remove any unbound ligands from the membranes before taking data. Carboxyl-dye conjugation Membranes of carboxyl-terminated ligands were first prepared as described above. Subsequently, concentrated stock solutions of the carboxyl-specific dye, Cascade Blue (LifeTechnologies) were prepared in water (~20 mg ml −1 ), and diluted down into an appropriate buffer that ranged from 1 to 150 mM NaCl, 1 to 10 mM NaHCO 3 , pH=7–10. The membranes were then immersed in a particular dye solution for ~1 h. Repeated washing with water, and flushing with the peristaltic pumping system, were used in conjunction with conductivity measurements to ensure any unbound dye molecules were removed before taking data. Conductivity rejections and corresponding charge densities were obtained at a fixed concentration of 5 mM NaCl. For the average values listed in the text, error bars correspond to s.d.’s in the fitted charge density for two different membranes. Experimental set-up Once assembled, membranes were incorporated into a peristaltic pump system composed of a modified Swinnex filter holder, teflon o-rings and a steel mesh for support (Millipore). The Swinnex filter holder was used inverted to its intended use and modified using a needle to introduce inlet and outlet valves. The inlet valve (1 mm diameter) was positioned 5 mm above the membrane surface and the outlet valve (1 mm diameter) on the side, 1.0 mm above the membrane. Flow was introduced in a direction perpendicular to the membrane surface via a peristaltic pump with a variable pump setting (MightyFlex, Model no. 913). Pump settings were calibrated for corresponding cross-flow velocities in the range 2 m s −1 (lowest setting) and 6 m s −1 . The presence of a cross-flow was required to mitigate concentration polarization that would affect ionic rejection. Concentrated salt solutions (~500 mM) were diluted into 1 l of feed solution until a desired concentration was reached, and all solutions were prepared using 0.22-μm pre-filtered 18-MΩ cm distilled water (Millipore). Conductivity differences between the feed and permeate solutions were measured using a Horiba meter (model B-171). Typical volumes of collected permeate were 40–100 μl, taken at random time intervals. At a given feed concentration, a series of six measurements on average was used to determine the conductivity rejection. Random samplings between different concentrations showed no difference from when the feed concentration was increased incrementally so that most concentration data (for example, Fig. 3 ) were obtained by incrementally increasing the concentration of salt in the feed solutions. Ionic conductivities were used as a measure of ionic concentration throughout. During salt tests of different ions, flow rate and the rejection of 1 mM NaCl were monitored to ensure that no noticeable changes to the membranes occurred (for example, fouling and/or specific adsorption of ions). All membranes studied under these conditions showed no signs of hysteresis over the tested ranges in salt concentration and pH. Membrane structural parameters High-flux characteristics, corresponding to permeabilities of L p ~(10 −9 –10 −10 ) m s −1 Pa −1 , were measured for dDT–AuNP-modified PC substrates with a pore diameter of 100 nm under pump-free conditions by measuring the flow rate (10–100 μl min −1 ) under a known pressure differential (~83 kPa). Permeabilities were calculated using the diameter of the membranes after accounting for the teflon o-ring (10 mm) and the steel mesh porosity (25%). How to cite this article: Barry, E. et al. Ion transport controlled by nanoparticle-functionalized membranes. Nat. Commun. 5:5847 doi: 10.1038/ncomms6847 (2014).